Interfacial assembly of protein–polymer nano-conjugates into stimulus-responsive biomimetic protocells The mechanism of spontaneous assembly of microscale compartments is a central question for the origin of life, and has technological repercussions in diverse areas such as materials science, catalysis, biotechnology and biomedicine. Such compartments need to be semi-permeable, structurally robust and capable of housing assemblages of functional components for internalized chemical transformations. In principle, proteins should be ideal building blocks for the construction of membrane-bound compartments but protein vesicles with cell-like properties are extremely rare. Here we present an approach to the interfacial assembly of protein-based micro-compartments (proteinosomes) that are delineated by a semi-permeable, stimulus-responsive, enzymatically active, elastic membrane consisting of a closely packed monolayer of conjugated protein–polymer building blocks. The proteinosomes can be dispersed in oil or water, thermally cycled to temperatures of 70 °C, and partially dried and re-inflated without loss of structural integrity. As a consequence, they exhibit protocellular properties such as guest molecule encapsulation, selective permeability, gene-directed protein synthesis and membrane-gated internalized enzyme catalysis. The design and construction of compartmentalized ensembles for modelling complex biological systems, exploring the origin of life, and advancing future living technologies is attracting considerable interest in a wide range of research communities [1] , [2] , [3] , [4] , [5] , [6] , [7] , [8] , [9] . Artificial cell-like architectures have been developed based on phospholipid vesicles [10] , [11] , [12] , [13] , [14] , [15] , polymersomes [16] , [17] , polymeric [18] , [19] , [20] or polypeptide capsules [21] , [22] , organic [23] , [24] , [25] , [26] and inorganic colloidosomes [27] , [28] , dendrimersomes [29] multi-compartment vesicles [30] , [31] , [32] and membrane-free peptide (polymer)/nucleotide micro-droplets (coacervates) [33] , [34] , [35] . In contrast, there are few reports on the use of protein-based building blocks as structural and functional modules for the spontaneous self-assembly of biomimetic protocells even though the intrinsic biocompatibility, biodegradability and biofunctionality of protein membranes offer important advantages. Recently, sacrificial inorganic nanoparticle templates have been coated with proteins using the layer-by-layer technique to obtain microscale capsules [36] , [37] , [38] ; however, these methods are experimentally laborious, use of the solid template core considerably lowers the encapsulation efficiency, and relatively harsh conditions have to be employed to etch out the nanoparticle template before obtaining the hollow structure. It therefore remains a considerable challenge to establish facile routes to water-filled protein-based vesicles and capsules that are distinguished by spontaneous processes of supramolecular self-assembly and high encapsulation efficiencies of functional components. In this regard, ‘giant amphiphiles’ based on protein–polymer conjugates with well-defined compositions have been recently prepared by chemical coupling or co-factor reconstitution methods, and shown to self-aggregate into various nanostructures such as rod-shaped micelles and sub-micrometre-sized vesicles [39] , or nanoparticles [40] . In a few instances, the protein–polymer conjugates have been used as emulsion stabilizers [41] , [42] . Inspired by this work, here we prepare amphiphilic protein–polymer constructs that exhibit temperature-responsive properties and display self-assembly behaviour at water droplet/oil interfaces to produce novel microscale compartments that are delineated by a semi-permeable membrane consisting of a closely packed monolayer of conjugated protein–polymer building blocks. We refer to these micro-compartments as ‘proteinosomes’ by analogy with colloidosomes [23] , and demonstrate how they can be used for the design and construction of stimulus-responsive biomimetic protocells capable of guest molecule encapsulation, selective permeability, gene-directed protein synthesis and membrane-gated enzyme catalysis. Protein–polymer nano-conjugates and proteinosome assembly A three-step procedure was used to prepare proteinosomes by interfacial assembly at the water droplet/oil interface of a Pickering emulsion ( Fig. 1 ). Hybrid-building blocks in the form of discrete protein–polymer nano-conjugates were synthesized by reaction of a mercaptothiazoline-activated terminal amide in the temperature-responsive polymer poly( N -isopropylacrylamide) (PNIPAAm, M n 8,800 g mol −1 , PDI 1.19, monomer repeat units=75; Supplementary Methods and Supplementary Figs S1–S4 ) with surface primary amine groups of cationized proteins such as bovine serum albumin (BSA-NH 2 , Supplementary Figs S5–S7 and Supplementary Table S1 ), myoglobin or haemoglobin. Formation of the protein–polymer building blocks was confirmed by the absence of discrete free protein bands in the SDS–PAGE gels compared with native BSA or BSA-NH 2 ( Fig. 2a ), a change in the zeta potential values from −22 to +13 to +9 mV for native BSA, BSA-NH 2 or BSA-NH 2 /PNIPAAm conjugates, respectively ( Fig. 2b ), and appropriate molecular weight differences in the MALDI-TOF MS profiles of BSA-NH 2 /PNIPAAm, which were consistent with the presence of at least three PNIPAAm chains per BSA molecule ( Fig. 2c ). The latter was consistent with ultraviolet–vis spectroscopy measurements, which gave an average value of 3.3 PNIPAAm chains per BSA molecule ( Supplementary Fig. S8 and Supplementary Table S2 ). DLS measurements of aqueous solutions of BSA, BSA-NH 2 or BSA-NH 2 /PNIPAAm conjugates at 20 °C gave mean hydrodynamic diameters by volume of 2.0, 2.0 and 3.1 nm, respectively, indicating an ~1.1 nm increase in size due to the presence of the covalently linked PNIPAm chains ( Supplementary Fig. S9 ). In contrast, the hydrodynamic diameter of the aqueous BSA-NH 2 /PNIPAAm conjugates measured at 40 °C, that is, above the lower critical solution temperature ( ca. 32 °C) of the polymer was 39.0 nm. We attribute the large increase in size to aggregation of the protein–polymer conjugates in water due to the increase hydrophobicity associated with the collapsed PNIPAm chains above the critical temperature. 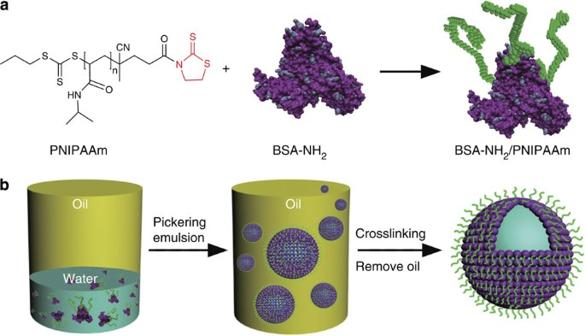Figure 1: General procedure for preparation of proteinosomes. (a) coupling of mercaptothiazoline-activated PNIPAAm polymer chains with primary amine groups of cationized BSA-NH2to produce protein–polymer nano-conjugates (BSA-NH2/PNIPAAm). The number of accessible amine groups available on the protein surface for coupling with the activated polymer, as well as for post-synthetic cross-linking, was enhanced by carbodiimide-activated cationization of aspartic and glutamic acid residues using 1,6-hexanediamine. Coupling reactions using native BSA and the mercaptothiazoline-activated PNIPAAm produced only very low yields of a protein–polymer conjugate. MALDI-TOF MS indicated that BSA-NH2consisted ofca.33 primary hexylamine groups per molecule, giving a total number ofca.60 surface accessible amines. The end-capped mercaptothiazoline-activated PNIPAAm was synthesized by reversible addition–fragmentation chain-transfer (RAFT) polymerization using a designed trithiol RAFT agent. (b) Use of protein–polymer building blocks for the spontaneous assembly of proteinosome micro-compartments in oil, and their transfer into a bulk water phase. An aqueous suspension of the amphiphilic, amide-coupled BSA-NH2/PNIPAAm nano-conjugates, along with functional components such as genes, ribosomes, nucleotides, amino acids, enzymes, proteins and inorganic nanoparticles, were emulsified in a continuous oil phase. Various oils were tested, and 2-ethyl-1-hexanol was generally used as it exhibited low volatility and immiscibility in water, and was a good solvent for PNIPAAm. As a consequence, the aqueous micro-droplets were stabilized by a self-assembled monolayer of closely packed protein–polymer nano-conjugates, which was then cross-linked using PEG-bis(N-succinimidyl succinate) (Mw2,000) into a continuous membrane at the oil/water droplet interface, and transferred into aqueous solutions by removal of the oil layer followed by dialysis using a series of water/ethanol mixtures. Proteinosome assembly did not occur in the presence of the unmodified protein, indicating that the amphiphilicity of the protein–polymer construct was critical for stabilizing the water micro-droplets. Figure 1: General procedure for preparation of proteinosomes. ( a ) coupling of mercaptothiazoline-activated PNIPAAm polymer chains with primary amine groups of cationized BSA-NH 2 to produce protein–polymer nano-conjugates (BSA-NH 2 /PNIPAAm). The number of accessible amine groups available on the protein surface for coupling with the activated polymer, as well as for post-synthetic cross-linking, was enhanced by carbodiimide-activated cationization of aspartic and glutamic acid residues using 1,6-hexanediamine. Coupling reactions using native BSA and the mercaptothiazoline-activated PNIPAAm produced only very low yields of a protein–polymer conjugate. MALDI-TOF MS indicated that BSA-NH 2 consisted of ca. 33 primary hexylamine groups per molecule, giving a total number of ca. 60 surface accessible amines. The end-capped mercaptothiazoline-activated PNIPAAm was synthesized by reversible addition–fragmentation chain-transfer (RAFT) polymerization using a designed trithiol RAFT agent. ( b ) Use of protein–polymer building blocks for the spontaneous assembly of proteinosome micro-compartments in oil, and their transfer into a bulk water phase. An aqueous suspension of the amphiphilic, amide-coupled BSA-NH 2 /PNIPAAm nano-conjugates, along with functional components such as genes, ribosomes, nucleotides, amino acids, enzymes, proteins and inorganic nanoparticles, were emulsified in a continuous oil phase. Various oils were tested, and 2-ethyl-1-hexanol was generally used as it exhibited low volatility and immiscibility in water, and was a good solvent for PNIPAAm. As a consequence, the aqueous micro-droplets were stabilized by a self-assembled monolayer of closely packed protein–polymer nano-conjugates, which was then cross-linked using PEG-bis( N -succinimidyl succinate) ( M w 2,000) into a continuous membrane at the oil/water droplet interface, and transferred into aqueous solutions by removal of the oil layer followed by dialysis using a series of water/ethanol mixtures. Proteinosome assembly did not occur in the presence of the unmodified protein, indicating that the amphiphilicity of the protein–polymer construct was critical for stabilizing the water micro-droplets. 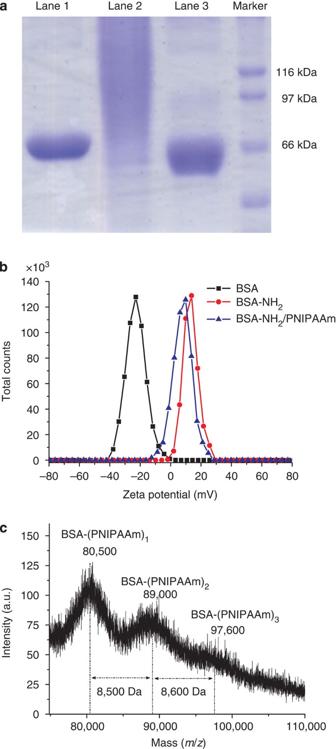Figure 2: Characterization of BSA-NH2/PNIPAAm conjugates. (a) SDS–PAGE profiles; lane 1, BSA-NH2; lane 2, BSA-NH2/PNIPAAm; lane 3, native BSA; and marker lane. (b) Zeta potential measurements for BSA (black, −22 mv), BSA-NH2(red, +13 mv) and BSA-NH2/PNIPAAm (blue, +9 mv) in 5.0 mM PBS pH 6.8 buffer solution at room temperature. (c) MALDI-TOF MS of BSA-NH2/PNIPAAm conjugates showing mass peaks for BSA conjugated with one, two or three PNIPAAm chains. The mass differences between neighbouring peaks correspond to the molecular weight of the synthesized PNIPAAm (Mn8,800 g mol−1, PDI 1.19). Full size image Figure 2: Characterization of BSA-NH 2 /PNIPAAm conjugates. ( a ) SDS–PAGE profiles; lane 1, BSA-NH 2 ; lane 2, BSA-NH 2 /PNIPAAm; lane 3, native BSA; and marker lane. ( b ) Zeta potential measurements for BSA (black, −22 mv), BSA-NH 2 (red, +13 mv) and BSA-NH 2 /PNIPAAm (blue, +9 mv) in 5.0 mM PBS pH 6.8 buffer solution at room temperature. ( c ) MALDI-TOF MS of BSA-NH 2 /PNIPAAm conjugates showing mass peaks for BSA conjugated with one, two or three PNIPAAm chains. The mass differences between neighbouring peaks correspond to the molecular weight of the synthesized PNIPAAm ( M n 8,800 g mol −1 , PDI 1.19). Full size image Mixing an aqueous solution of BSA-NH 2 /PNIPAAm (0.2–10 mg ml −1 ) with 2-ethyl-1-hexanol at an aqueous/oil volume fraction ( φ w ) of 0.06 produced a dispersion of proteinosomes that sedimented within 1 h to give a turbid water-in-oil emulsion lower phase and a transparent upper oil layer. The proteinosomes were in the form of hollow spherical microstructures with diameters in the range of 20–50 μm ( Fig. 3a ), and were structurally stable and remained non-aggregated at room temperature over several weeks. Similar results were obtained for proteinosomes prepared using building blocks based on synthesized myoglobin-NH 2 /PNIPAAm or haemoglobin-NH 2 /PNIPAAm nano-conjugates ( Supplementary Figs S10 and S11 ), suggesting that the methodology was versatile. The hollow architecture was clearly visible in optical images of partially dried proteinosomes, which showed a collapsed but intact structure ( Fig. 3b ). Scanning electron microscope ( Fig. 3c ), transmission electron microscopy ( Fig. 3d ) and cryo-transmission electron microscopy ( Fig. 3e and Supplementary Fig. S12 ) images of the micro-compartments indicated that the BSA-NH 2 /PNIPAAm shell consisted of a flexible ultra-thin membrane that was structurally robust when dried under vacuum. Based on AFM measurements, the thickness of the proteinosome membrane was determined as ca. 10 nm ( Fig. 3f,g ). Given that the theoretical extended length of a BSA-NH 2 /PNIPAAm molecule was around 9 nm, the similarity between the thickness of the membrane and the maximum length of the building block suggested that the proteinosome membrane was composed of single layer of the BSA-NH 2 /PNIPAAm conjugate. Interestingly, the average diameter of the proteinosomes could be systematically controlled between 10 and 200 μm by changing the concentration of the BSA-NH 2 /PNIPAAm conjugate at a constant φ w value of 0.06 ( Fig. 3h ). Increasing the concentration of the protein–polymer building blocks from 0.2 to 8 mg ml −1 resulted in a monotonic reduction in the mean size of the micro-compartments ( Supplementary Fig. S13 ). This was consistent with stabilization of the increased oil/water interfacial area associated with smaller water droplets in the presence of increasing amounts of the amphiphilic protein–polymer nano-conjugates. 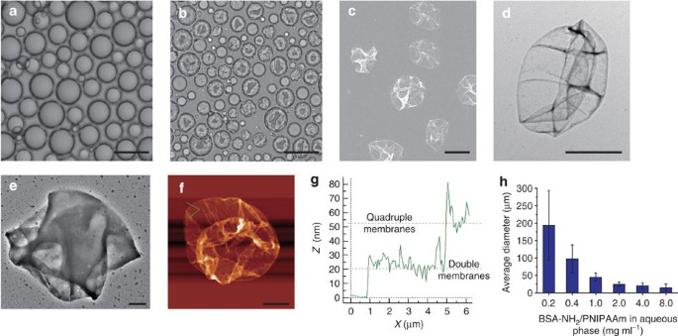Figure 3: Structural and morphological characterization of proteinosomes. (a,b) Optical microscopy images of proteinosomes dispersed in oil (a), or after partial drying in air (b). (c) Scanning electron microscope (SEM), (d) transmission electron microscope (TEM) and (e) cryo-TEM images showing continuous and flexible proteinosome membranes. (f) Atomic force microscopy (AFM) image of a dried proteinosome and (g) corresponding height profile along the green trace (upper, left corner) that traverses both double and quadruple membrane thicknesses associated with the collapsed/folded sample. (h) Plot showing mean size (bars) and s.d. (lines on bars) of proteinosomes dispersed in oil and prepared at different concentrations of BSA-NH2/PNIPAAm between 0.2–8.0 mg ml−1atφw=0.06. Scale bars ina–fare 50, 50, 10, 5, 0.5 and 5 μm, respectively. Figure 3: Structural and morphological characterization of proteinosomes. ( a , b ) Optical microscopy images of proteinosomes dispersed in oil ( a ), or after partial drying in air ( b ). ( c ) Scanning electron microscope (SEM), ( d ) transmission electron microscope (TEM) and ( e ) cryo-TEM images showing continuous and flexible proteinosome membranes. ( f ) Atomic force microscopy (AFM) image of a dried proteinosome and ( g ) corresponding height profile along the green trace (upper, left corner) that traverses both double and quadruple membrane thicknesses associated with the collapsed/folded sample. ( h ) Plot showing mean size (bars) and s.d. (lines on bars) of proteinosomes dispersed in oil and prepared at different concentrations of BSA-NH 2 /PNIPAAm between 0.2–8.0 mg ml −1 at φ w =0.06. Scale bars in a – f are 50, 50, 10, 5, 0.5 and 5 μm, respectively. Full size image Transfer of cross-linked proteinosomes into a continuous water phase was achieved without loss of structural integrity. Significantly, the transferred proteinosomes could be partially air-dried to produce shrunken, collapsed shells, which could be rapidly inflated by rehydration into intact hollow micro-architectures ( Supplementary Fig. S14 ). The results indicated that the cross-linked protein–polymer membrane was elastic and robust under these conditions. Bright-field optical microscopy images of the transferred proteinosomes were generally low in contrast ( Fig. 4a ). To circumvent this, we prepared and transferred into water BSA-NH 2 /PNIPAAm proteinosomes incorporating a fluorescence dye-labelled PNIPAAm (fluorescein O -methacrylate (FOMA)-PNIPAAm), which was synthesized by using fluorescein O -methacrylate as a co-monomer during the polymerization process. The corresponding fluorescence microscopy images showed the presence of green fluorescence associated specifically with the intact micro-compartments ( Fig. 4b ), confirming that the polymer remained covalently attached to the proteinosome membrane after cross-linking and transfer into water. Furthermore, measurements of individual water-dispersed proteinosomes that were thermally cycled from below (25 °C) to above (40 °C) the lower critical solution temperature ( ca. 32 °C) of the PNIPAAm polymer chains showed an ~4% reversible decrease/increase in the diameter of the micro-compartments ( Fig. 4c and Supplementary Fig. S15 ), indicating that PNIPAAm was both a structural and functional component of the protein–polymer membrane. 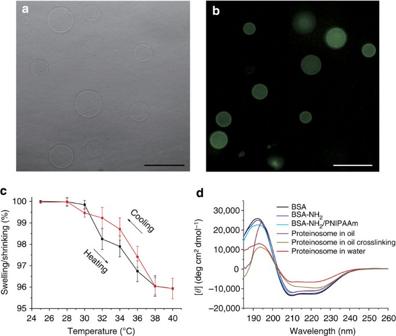Figure 4: Transfer of proteinosomes into water. (a) Optical microscopy image and (b) fluorescence microscopy image of BSA-NH2/PNIPAAm proteinosomes in aqueous solution; the fluorescence originates from fluorescein-labelled PNIPAAm (fluorescein isothiocyanate (FITC)-PNIPAAm) used to construct the protein–polymer building blocks; scale bar, 50 μm. (c) Plot showing temperature-induced changes in diameter for an individual proteinosome dispersed in aqueous solution; heating (black line) and cooling (red line) cycle is shown; error bars represent measurements from five single proteinosomes. (d) CD spectra for BSA, BSA-NH2, BSA-NH2/PNIPAAm, non-cross-linked or cross-linked BSA-NH2/PNIPAAm proteinosomes in oil, and cross-linked BSA-NH2/PNIPAAm proteinosomes dispersed in aqueous solution at room temperature. Figure 4: Transfer of proteinosomes into water. ( a ) Optical microscopy image and ( b ) fluorescence microscopy image of BSA-NH 2 /PNIPAAm proteinosomes in aqueous solution; the fluorescence originates from fluorescein-labelled PNIPAAm (fluorescein isothiocyanate (FITC)-PNIPAAm) used to construct the protein–polymer building blocks; scale bar, 50 μm. ( c ) Plot showing temperature-induced changes in diameter for an individual proteinosome dispersed in aqueous solution; heating (black line) and cooling (red line) cycle is shown; error bars represent measurements from five single proteinosomes. ( d ) CD spectra for BSA, BSA-NH 2 , BSA-NH 2 /PNIPAAm, non-cross-linked or cross-linked BSA-NH 2 /PNIPAAm proteinosomes in oil, and cross-linked BSA-NH 2 /PNIPAAm proteinosomes dispersed in aqueous solution at room temperature. Full size image The presence of BSA in the transferred proteinosomes was confirmed by circular dichroism (CD) spectroscopy ( Fig. 4d ). The spectra showed minimal changes in the characteristic peak intensities at 222 and 208 nm for native BSA, BSA-NH 2 , aqueous BSA-NH 2 /PNIPAAm conjugates or BSA-NH 2 /PNIPAAm proteinosomes dispersed in oil, indicating that polymer conjugation and interfacial self-assembly was achieved without significant disruption to the predominantly α-helical protein secondary structure. In contrast, a decrease in the peak intensities was observed after cross-linking the BSA-NH 2 /PNIPAAm proteinosomes in oil, and after transfer into water ( Fig. 4d ). These changes were attributed to reaction of the PEG-bis( N -succinimidyl succinate) cross-linker with primary amine groups on the surface of BSA as well as exposure to ethanol during the phase transfer process. Deconvolution of the CD spectra showed that the level of α-helical secondary structure in the aqueous dispersed cross-linked proteinosome membrane was 36% compared with 66% in BSA-NH 2 /PNIPAAm, and that this was associated with an increase in the content of the β-sheet, turn and unordered domains from 10%, 12% and 13% to 22%, 17% and 26%, respectively (see Supplementary Table S3 ). Based on the above changes in secondary structure, we tested the esterase activity of the BSA-NH 2 /PNIPAAm proteinosomes in oil and water. Surprisingly, although covalent grafting of the PNIPAAm chains onto the surface of BSA-NH 2 produced an ~30% reduction in the esterase activity, interfacial assembly of the proteinosomes in oil, cross-linking with PEG-bis( N -succinimidyl succinate) or transfer into water did not lead to any further decreases in enzyme activity ( Supplementary Fig. S16 ). As a consequence, proteinosomes with enzymatically active, structurally robust membranes could be prepared in both oil or water continuous phases. Protocell properties Given the above observations, we explored the use of the BSA-NH 2 /PNIPAAm micro-compartments as a step towards preparing synthetic protocells with a range of biomimetic properties, including guest molecule encapsulation, selective permeability, protein synthesis via gene expression, and membrane-gated internalized enzyme catalysis. Encapsulation of a wide range of functional components such as small-molecule fluorescence dyes (calcein, rhodamine 6G (Rh6G)), drug molecules (doxorubicin), proteins (myoglobin, ferritin), enzymes (RNA polymerases, alkaline phosphatase (ALP) and lipoprotein lipase (LPL)) and inorganic nanoparticles of various sizes (gold (15 nm), silica (500 nm)) was readily achieved using the above preparation procedure ( Fig. 5a,b , and Supplementary Figs S17 and S18 ). In some cases, high concentrations could be entrapped; for example, micro-compartments with 15 mg ferritin per 1 mg proteinosomes could be readily prepared in the oil phase. Significantly, it was possible to encapsulate the hundred or so components of a cell-free expression system, including ribosomes, tRNA, transcription and translation co-factors, reaction buffer, nucleotides for mRNA synthesis, amino acids for translation and an ATP regeneration system to prolong and sustain gene expression. As a consequence, we were able to successfully undertake gene-directed protein synthesis in non-cross-linked BSA-NH 2 /PNIPAAm proteinosomes dispersed in oil. For example, the in vitro expression of enhanced green fluorescent protein (eGFP) was undertaken by constructing a plasmid DNA vector pEXP5-NT/eGFP using polymerase chain reaction procedures (see Supplementary Methods ), and adding the plasmid to the cell-free gene expression solution before formation of the proteinosomes ( Fig. 5c ). Optical microscopy images showed well-defined proteinosomes, 50–150 μm in diameter ( Fig. 5d ), and significantly, in vitro synthesis of eGFP specifically within the proteinosomes over a period of 2 h was confirmed by fluorescence microscopy ( Fig. 5e ). In contrast, only a weak background auto-fluorescence was observed at 520 nm in the absence of eGFP synthesis. Expression of eGFP both within the BSA-NH 2 /PNIPAAm micro-compartments and in bulk solution was monitored over time by changes in the fluorescence intensity at 516 or 510 nm using an excitation wavelength of 470 nm ( Supplementary Fig. S19 ); in both cases, the reaction profiles showed a similar quasi-exponential decrease in the rates of gene expression ( Fig. 5f ). 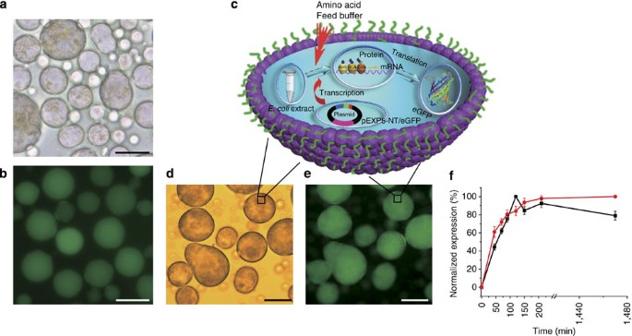Figure 5: Encapsulation andin vitrogene expression of eGFP in proteinosomes. (a,b) Optical/fluorescence microscopy images of proteinosomes dispersed in oil with encapsulated ferritin (a) or calcein (b); scale bar, 50 μm. The red coloration and green fluorescence originate from ferritin or calcein, respectively, entrapped within the micro-compartment interior. (c) Schematic illustration showing the procedure for cell-free gene expression of eGFP in proteinosomes. (d) Optical microscopy image showing proteinosomes containing plasmid pEXP5-NT/eGFP and a cell-free gene expression solution after 2 h incubation at 37 °C, and (e) corresponding fluorescence micrograph showing characteristic green fluorescence associated within vitrogene expression of eGFP after 2 h (scale bar, 100 μm). Samples were excited in blue light. (f) Plots showing expression profiles for eGFP in bulk solution (red line) and in proteinosomes (black line); error bars represent three repeat experiments. Figure 5: Encapsulation and in vitro gene expression of eGFP in proteinosomes. ( a , b ) Optical/fluorescence microscopy images of proteinosomes dispersed in oil with encapsulated ferritin ( a ) or calcein ( b ); scale bar, 50 μm. The red coloration and green fluorescence originate from ferritin or calcein, respectively, entrapped within the micro-compartment interior. ( c ) Schematic illustration showing the procedure for cell-free gene expression of eGFP in proteinosomes. ( d ) Optical microscopy image showing proteinosomes containing plasmid pEXP5-NT/eGFP and a cell-free gene expression solution after 2 h incubation at 37 °C, and ( e ) corresponding fluorescence micrograph showing characteristic green fluorescence associated with in vitro gene expression of eGFP after 2 h (scale bar, 100 μm). Samples were excited in blue light. ( f ) Plots showing expression profiles for eGFP in bulk solution (red line) and in proteinosomes (black line); error bars represent three repeat experiments. Full size image Transfer of the BSA-NH 2 /PNIPAAm proteinosomes into water resulted in retention of macromolecular guest components such as proteins and enzymes ( Fig. 6a–c and Supplementary Fig. S20 ), whilst small molecules such as Rh6G leached out into the continuous water phase within a few hours ( Fig. 6d,e and Supplementary Fig. S21 ). Uptake studies in the presence of fluorescent-labelled dextran indicated that the proteinosome membrane was essentially impermeable to the polysaccharide above a molecular weight cutoff of 40 kDa ( Supplementary Figs S22 and S23 ). These observations were consistent with diffusion-limited transfer associated with the intrinsic molecular scale permeability of the cross-linked protein–polymer membrane. Given this intrinsic porosity, and the ability of the proteinosome membrane to structurally respond to changes in temperature (see Fig. 4c ), we investigated whether diffusion of Rh6G molecules through the protein–polymer membrane could be influenced by thermally induced changes in the polymer conformation and hydrophobicity. Kinetic profiles for release of Rh6G in free solution through a dialysis membrane showed an approximate doubling in the rate of diffusion after 1 h at 40 °C compared with at room temperature ( Supplementary Fig. S24 ). In contrast, the rates of release of Rh6G were essentially the same after 1 h at 40 °C and room temperature when the cationic dye was encapsulated within the BSA-NH 2 /PNIPAAm proteinosomes in aqueous solution ( Supplementary Fig. S25 ). Given the considerable increase in release expected at 40 °C, the reduced rate of Rh6G efflux was consistent with an increase in hydrophobicity of the proteinosome membrane above the lower critical solution transition temperature of 33 °C. Analogous experiments undertaken with the drug molecule doxorubicin also showed similar rates above and below the lower critical solution transition temperature even though diffusion in the control experiments was markedly increased at 40 °C ( Supplementary Fig. S26 ). 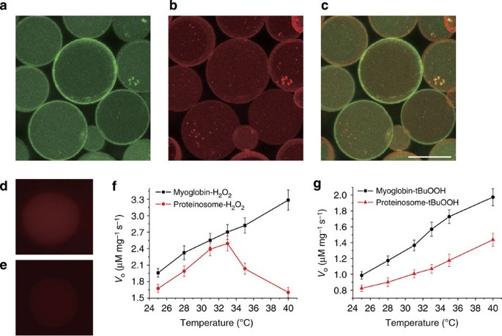Figure 6: Permeability and membrane-gated enzyme catalysis. (a–c) Confocal images of myoglobin-encapsulated, BSA-NH2/fluorescein isothiocyanate (FITC)-PNIPAAm proteinosomes in aqueous solution after 6 h showing retention of myoglobin after transfer into water, (a) green fluorescence corresponding to the FITC-PNIPAAm component of the proteinosome membrane, (b) red fluorescence associated with encapsulated myoglobin, which was covalently labelled with rhodamine B, and (c) corresponding overlay image; scale bar, 20 μm. (d,e) Fluorescence microscopy images of single Rh6G-encapsulated proteinosome images recorded 1 min (d) and 60 min (e) after transfer into water showing progressive efflux of the cationic dye into the continuous water phase. (f,g) Temperature-dependent catalytic reaction rates of free myoglobin (black lines) and proteinosome-encapsulated myoglobin (red lines) in the presence of 2-methoxyphenol (5 mM) and H2O2(20 mM) (f), or 2-methoxyphenol and tBuOOH (20 mM) (g); error bars represent three repeat experiments. Figure 6: Permeability and membrane-gated enzyme catalysis. ( a – c ) Confocal images of myoglobin-encapsulated, BSA-NH 2 /fluorescein isothiocyanate (FITC)-PNIPAAm proteinosomes in aqueous solution after 6 h showing retention of myoglobin after transfer into water, ( a ) green fluorescence corresponding to the FITC-PNIPAAm component of the proteinosome membrane, ( b ) red fluorescence associated with encapsulated myoglobin, which was covalently labelled with rhodamine B, and ( c ) corresponding overlay image; scale bar, 20 μm. ( d , e ) Fluorescence microscopy images of single Rh6G-encapsulated proteinosome images recorded 1 min ( d ) and 60 min ( e ) after transfer into water showing progressive efflux of the cationic dye into the continuous water phase. ( f , g ) Temperature-dependent catalytic reaction rates of free myoglobin (black lines) and proteinosome-encapsulated myoglobin (red lines) in the presence of 2-methoxyphenol (5 mM) and H 2 O 2 (20 mM) ( f ), or 2-methoxyphenol and tBuOOH (20 mM) ( g ); error bars represent three repeat experiments. Full size image Based on these observations, we undertook proof-of-principle experiments to demonstrate thermally induced gating of the membrane permeability to external substrates such that an enzymatic reaction rate inside the micro-compartments could be effectively switched on and off. To demonstrate this principle, myoglobin was used as a peroxidase and encapsulated within the BSA-NH 2 /PNIPAAm proteinosomes, which were subsequently transferred into water. The samples were centrifuged (MWCO 50 kDa filter) to remove any myoglobin released into the bulk water phase by fragmentation of the micro-compartments during transfer, and then hydrogen peroxide (H 2 O 2 ) and 2-methoxyphenol (guaiacol) were added to the bulk water phase as small-molecule substrates. Myoglobin-catalysed peroxidation of 2-methoxyphenol to produce the cyclic aromatic, tetraguaiacol, was monitored by recording the increase in absorbance at 470 nm of the proteinosome dispersion. At 25 °C, the catalytic reaction rate of the encapsulated myoglobin was 1.66 μM s −1 per mg myoglobin, which was very similar to the reaction rate of free myoglobin (1.96 μM s −1 per mg myoglobin) measured under the same conditions. Thus, at temperatures below the lower critical solution temperature of PNIPAAm, the expanded hydrated state of the proteinosome membrane was highly permeable to the substrate molecules, and no diffusional constraints were placed on the compartmentalized enzyme reaction. However, increasing the temperature from 25 up to 40 °C produced a progressive increase in the reaction rate for myoglobin in bulk solution, whilst the encapsulated enzyme showed an increase in rate up to a temperature of 33 °C followed by a rapid decrease ( Fig. 6f ). Indeed, at 40 °C the reaction rate was twice as fast in the continuous water phase compared with inside the proteinosomes, implying that peroxidase activity was effectively switched off in the latter system. Clearly, the reaction behaviour correlated strongly with the onset of the extended to folded polymer transition associated with the lower critical solution temperature of PNIPAAm. We therefore attributed the loss of enzymatic activity to diffusional constraints associated with a reduction in membrane pore size due to polymer deswelling or an increase in the hydrophobicity of the BSA-NH 2 /PNIPAAm shell, or both. To elucidate the possible mechanism, we used a small-molecule, partially hydrophobic substrate, tert-butyl hydroperoxide (tBuOOH), instead of H 2 O 2 , and determined the enzyme activities for free and proteinosome-encapsulated myoglobin. In contrast to the hydrophilic substrates, peroxidation of of 2-methoxyphenol by tBuOOH increased with temperature, albeit at a rate that was lower than for free myoglobin, and no evidence of a polymer transition-induced inhibition was observed above 33 °C ( Fig. 6g ). The results indicated that the BSA-NH 2 /PNIPAAm membrane remained semi-permeable to the partially hydrophobic substrate above the polymer transition, suggesting that the membrane-gated inhibition observed in the presence of H 2 O 2 above 33 °C was primarily associated with loss of hydrophilicity in the protein–polymer shell, although secondary factors such as the reduction in pore size associated with the coil to globule polymer chain transition could not be ruled out. We tested this hypothesis further by investigating the proteinosome-encapsulated activity of two other enzymes, ALP or LPL, in the presence of a hydrophilic ( p -nitrophenyl phosphate) or hydrophobic (4-nitrophenyl butyrate) substrate, respectively ( Supplementary Fig. S27 ). In both cases, the temperature-dependent kinetic profiles were consistent with hydrophobically mediated gating of the proteinosome membrane permeability in the presence of small-molecule substrates. The above results demonstrate that enzymatically active protein-based micro-compartments capable of guest molecule encapsulation, selective permeability and gene-directed protein synthesis can be spontaneously assembled from discrete, amphiphilic protein–polymer nano-conjugates. By using protein molecules as the basis for the hybrid building blocks, it should be possible to construct a diversity of functional micro-compartments with high levels of biocompatibility and cellular recognition, for use in the targeted delivery of a complementary suite of therapeutic agents, for example. Moreover, by covalently grafting PNIPAAm onto the protein surface temperature-dependent changes in the polymer chain conformation can be exploited to produce stimulus-responsive proteinosomes that exhibit self-mediated gated permeability at water/water phase boundaries. In principle, this offers the ability not only to produce targeted micro-containers but also to use localized cooling of targeted cells and tissues for the temperature-mediated release of bioactive payloads. More generally, the intrinsic elasticity of the protein–polymer membrane provides a robust, porous micro-architecture that can withstand partial dehydration and rehydration, suggesting that it should be possible to exploit proteinosomes for the sustained storage and release of a wide range of drug and bioactive agents. In this context, we also observed that proteinosomes dispersed in oil or water remained structurally intact when held at a temperature of 70 °C for 90 min ( Supplementary Figs S28 and S29 ), suggesting that they could also be exploited for applications requiring the microscale confinement of thermophilic enzymes or temperature cycling procedures, such as in the amplification of entrapped genetic material by PCR methods. Given the range of these multifunctional properties, we therefore expect proteinosomes to be useful in new micro-reactor technologies, as novel constructs for cytomimetic engineering, and as compartmentalized ensembles for diverse applications in synthetic biology and biomaterials research. Synthesis Carbodiimide-activated conjugation of 1,6-diaminohexane to aspartic and glutamic acid residues on the external surface of BSA was used to prepare the cationized protein, BSA-NH 2 . For this, a solution of 1,6-diaminohexane (1.5 g) was adjusted to pH 6.5 using 5 M HCl, and added dropwise to a stirred solution of BSA (200 mg). The coupling reaction was initiated by adding N -ethyl- N ′-(3-dimethylaminopropyl) carbodiimide hydrochloride (EDAC, 100 mg) immediately, and again (50 mg) after 5 h. The pH value was maintained at 6.5 using dilute HCl, and the solution was stirred for a further 6 h. The solution was then centrifuged to remove any precipitate and the supernatant dialysed (dialysis tubing 12–14 kDa MWCO) extensively against Milli-Q water. The final product was obtained by freeze-drying. On average, 33 primary amine groups were linked per BSA-NH 2 molecule. End-capped mercaptothiazoline-activated PNIPAAm ( Mn 8,800 g mol −1 , 10 mg in 5 ml of water; see Supplementary Methods for polymer synthesis details) was added to a stirred solution of BSA-NH 2 (10 mg, in 5 ml of PBS buffer pH 8.0) to give a polymer: protein molar ratio of ~9: 1. The mixed solution was stirred for 12 h, and then purified by using a centrifugal filter (MWCO 50 kDa) to remove any unreacted PNIPAAm and salts. After freeze-drying, the obtained BSA-NH 2 /PNIPAAm conjugate was characterized by SDS–PAGE, MALDI-MS, zeta potentiometry and ultraviolet–vis spectroscopy. Preparation of proteinosomes Proteinosomes were prepared by mixing an aqueous BSA-NH 2 /PNIPAAm solution with 2-ethyl-1-hexanol followed by shaking the mixture by hand for 10 s. The samples were prepared at a constant aqueous/oil volume fraction ( φ w ) of 0.06. Typically, 0.06 ml of aqueous BSA-NH 2 /PNIPAAm (4.0 mg ml −1 , pH 8.5, sodium carbonate buffer) were mixed with 1.0 ml of the oil. The proteinosomes were then cross-linked in the continuous oil phase by addition of PEG-bis( N -succinimidyl succinate) (0.5 mg), which reacted with free primary amine groups of BSA-NH 2 . Transfer of the cross-linked proteinosomes into water was achieved as follows. After 3 h sedimentation, the upper clear oil layer was discarded and 1 ml of 65% ethanol was added and the emulsion gently shaken. The dispersion was then dialysed against 65% ethanol for 5 h, 50% ethanol for 2 h, 30% ethanol for 2 h and milli-Q water for 2 days to complete the phase transfer process. Proteinosomes comprising encapsulated components including metal ions (Cu(NO 3 ) 2 ), dyes (calcein, Rh6G), proteins and enzymes (ferritin, myoglobin, ALP and LPL), a cell-free gene expression kit or inorganic nanoparticles (gold (15 nm), silica (500 nm)) were prepared following the above procedures except that the encapsulants were added to the aqueous BSA-NH 2 /PNIPAAm solution before mixing with the oil phase. In vitro gene expression Cell-free gene expression of eGFP from pEXP5-NT/eGFP was undertaken using an in vitro gene expression system (Expressway Cell-Free E. coli Expression System, Invitrogen) comprising S30 E. coli extract, reaction buffer, proprietary T7 enzyme mix, amino acid (-Met) mixture and methionine solution. The kit was used according to the manufacturer’s instructions unless otherwise stated. Typically, 20 μl of S30 E. coli extract, 20 μl of the reaction and feed buffers, 1 μl of proprietary T7 enzyme mix, 1.25 μl of a 50 mM amino acid (-Met) mixture, 1 μl of 75 mM methionine solution and 789 ng of pEXP5-NT/eGFP were mixed together, made up to a final volume of 50 μl with DNAase/RNAse-free water, and incubated in a 1.5 ml PCR-ready, sterile centrifuge tube at 37 °C for 30 min. After incubation, a feed solution containing 25 μl of feed buffer, 2.5 μl of 50 mM amino acid (-Met) mixture, 2 μl of 75 mM methionine solution and 20.5 μl of DNAase/RNAse-free water was added to the extract/reaction mixture, which was gently homogenized by tapping the side of the vial to produce an in vitro gene expression solution with a final volume of 100 μl. A 30 μl aliquot of the aqueous in vitro gene expression solution was mixed with 30 μl of aqueous BSA-NH 2 /PNIPAAm (4.0 mg ml −1 ) with gentle shaking, followed by addition of 1.0 ml of 2-ethyl-1-hexanol and shaking by hand for 5 s. The resulting emulsion was then incubated at 37 °C. In vitro gene expression of eGFP was monitored on individual droplets by using bright-field optical and fluorescence (excitation 450–490 nm) microscopies. Protein synthesis was also monitored by measuring the time-dependent change in fluorescence intensity at 520 nm using an excitation wavelength of 470 nm (Jasco FP-6500 spectrofluorometer). Release behaviour of Rh6G Rh6G was encapsulated into the proteinosome aqueous interior by adding 20 μl of 1.0 mM Rh6G aqueous solution to 40 μl of BSA-NH 2 /PNIPAAm (4.0 mg ml −1 ) solution, followed by addition of 1.0 ml of 2-ethyl-1-hexanol. The proteinosomes were then cross-linked and transferred into water as described above. The aqueous dispersion of Rh6G-containing proteinosomes was dispersed into 20 ml of Milli-Q water and divided in half by volume, and either stirred at room temperature, or stirred at 40 °C. Rh6G release was measured by monitoring the decrease in Rh6G concentration in individual proteinosomes by recording the fluorescence intensity using fluorescence microscopy. In addition, ultraviolet–vis spectroscopy was used to record the released Rh6G after filtering 1 ml of the proteinosome bulk solution; the release kinetics were plotted as a percentage of the maximum ultraviolet–vis absorbance (530 nm) against time. Monitoring was undertaken immediately on transfer into water although some loss of the dye inevitably occurred during the transfer process procedures. Control experiments were undertaken in which the rates of transfer of free Rh6G through a dialysis membrane at room temperature and 40 °C were determined. Enzyme activity within proteinosomes Studies on enzyme-mediated reactions in proteinosomes were carried out by encapsulating myoglobin, ALP or LPL. Typically, 30 μl of myoglobin solution (1 mg ml −1 , in pH 7.4, 5 mM PBS buffer) and 30 μl of BSA-NH 2 /PNIPAAm (4.0 mg ml −1 ) were mixed with gentle shaking, then 1.0 ml of 2-ethyl-1-hexanol was added, and the mixture shaken by hand for 5 s followed by addition of the PEG-bis( N -succinimidyl succinate) (Mw 2,000, 0.5 mg) cross-linker. After 5 h, the upper clear oil layer was removed and the cross-linked proteinosome with encapsulated myoglobin was transferred into water. The final solution was further purified by using a centrifugal filter (MWCO 50 kDa) to remove any free myoglobin. The enzyme reaction rate was monitored by ultraviolet–vis spectroscopy at 470 nm using a 500 μl quartz cuvette containing 100 μl of myoglobin-encapsulated proteinosomes. The reaction was initiated by addition of 100 μl of 0.025 M 2-methoxyphenol (guaiacol), 100 μl of 0.1 M H 2 O 2 and 200 μl of pH 7.4, 100 mM PBS buffer to the continuous water phase. The enzyme reaction within the proteinosomes was monitored for 300 s. The initial catalytic reaction rate was calculated based on the following equation: [ V 0 ]=Δ A /(Δ t × ε × b × [ E 0 ]), where, Δ A /(Δ t was the initial change of absorbance with time, ε the extinction coefficient of the brown product (tetraguaiacol: 26,600 M −1 cm −1 ), [ E 0 ] the concentration of the enzyme in the proteinosome, and b the path length of the quartz cuvette (1 cm). Similar studies of enzyme activity within the proteinosomes were undertaken in the presence of encapsulated ALP or LPL. In the former case, 100 μl of 0.025 M p -nitrophenyl phosphate (substrate) and 300 μl of pH 8.8, 100 mM Tris buffer solution (containing 1 mM MgCl 2 ) was added to the continuous water phase of 100 μl of ALP-encapsulated proteinosomes. The reaction within the proteinosomes was monitored by ultraviolet–vis spectroscopy at 400 nm for 300 s, and the catalytic reaction rate determined using the extinction coefficient of the product p -nitrophenolate (17,500 M −1 cm −1 ) at pH 8.8 in Tris buffer. For the LPL-encapsulated micro-compartments, 100 μl of 5 mM p -nitrophenyl butyrate (substrate; prepared in 40% acetonitrile aqueous solution) and 300 μl of pH 7.4, 100 mM PBS buffer solution were added to the continuous water phase of 100 μl of the proteinosome suspension. The reaction was monitored by ultraviolet–vis spectrometer at 400 nm for 300 s, and the catalytic reaction rate determined using the extinction coefficient of the p- nitrophenolate product (12,000 M −1 cm −1 ) in pH 7.4 PBS buffer. How to cite this article: Huang X. et al. Interfacial assembly of protein–polymer nano-conjugates into stimulus-responsive biomimetic protocells. Nat. Commun. 4:2239 doi: 10.1038/ncomms3239 (2013).